Humans display a ‘cooperative phenotype’ that is domain general and temporally stable Understanding human cooperation is of major interest across the natural and social sciences. But it is unclear to what extent cooperation is actually a general concept. Most research on cooperation has implicitly assumed that a person’s behaviour in one cooperative context is related to their behaviour in other settings, and at later times. However, there is little empirical evidence in support of this assumption. Here, we provide such evidence by collecting thousands of game decisions from over 1,400 individuals. A person’s decisions in different cooperation games are correlated, as are those decisions and both self-report and real-effort measures of cooperation in non-game contexts. Equally strong correlations exist between cooperative decisions made an average of 124 days apart. Importantly, we find that cooperation is not correlated with norm-enforcing punishment or non-competitiveness. We conclude that there is a domain-general and temporally stable inclination towards paying costs to benefit others, which we dub the ‘cooperative phenotype’. Cooperation is fundamental to the success of social species. Yet cooperation requires individuals to bear costs to benefit others. Understanding how and when humans cooperate, as well as why evolution and strategic reasoning would give rise to cooperation, is therefore a major challenge for researchers across the natural and social sciences. To that end, recent years have seen a great deal of theoretical [1] , [2] , [3] , [4] , [5] , [6] and empirical [7] , [8] , [9] , [10] , [11] , [12] investigations of cooperation. This body of work has been particularly shaped by game theory: a number of simple games have been proposed that capture different facets of the tension between individual and collective interests, such as the Public Goods Game (PGG), the Trust Game (TG) and the Dictator Game (DG) (for a review, see ref. 9 ). Theoretical models ask which strategies in a given game will be favoured by natural selection, or chosen by players with particular preferences. Behavioural experiments explore how sets of rules affect actual decisions. Based on the results, researchers draw general conclusions about human prosociality. Beneath these conclusions lies a fundamental assumption: that decisions in cooperation games reflect a domain-general tendency towards prosociality. If behaviour in one game has little to do with behaviour in another (or with behaviour at a later date), then drawing broader conclusions from experimental findings becomes difficult. If this was the case, such laboratory games would not be a useful model of real-world cooperation [13] . Despite the centrality of this assumption, however, it is rarely acknowledged. Even more importantly, there is surprisingly little experimental evidence in support of a domain-general penchant for cooperation. Here we make this assumption explicit, and introduce the term ‘cooperative phenotype’ to describe it. We then generate a large body of experimental data supporting the existence of this cooperative phenotype. We begin by asking whether play correlates across different cooperation games. We also ask whether play in these games predicts play in other, potentially theoretically related, social games: norm-enforcing punishment games and competition games. Next, we ask whether game play reflects underlying moral values, as well as actual helping behaviour outside of economic games. Finally, we assess how stable an individual’s play in games is across time. Taken together, our experiments provide an extensive assessment of the domain generality of human social preferences, providing compelling evidence of a ‘cooperative phenotype’. Correlations between games To examine correlations in play across games, and between game play and self-reported values and behaviour, we recruit N =576 individuals from the United States to participate in an online experiment using Amazon Mechanical Turk [14] (see Methods for a discussion of the validity of data gathered using this platform). Participants make a total of eight different one-shot economic game decisions, in random order. We include four decisions that involve helping others: the PGG, the DG, and both roles in the TG (TG1 and TG2). These games vary in their specifics, but all involve paying a personal cost to give a benefit to one or more others (although note that in TG1 paying this cost may ultimately be payoff-maximizing depending on the choice of the other player). Thus, if a cooperative phenotype exists, we expect an individual’s behaviour across these games to be correlated. See Fig. 1a for a description of each cooperation game (note that in TG, TG1 corresponds to player A while TG2 corresponds to player B). 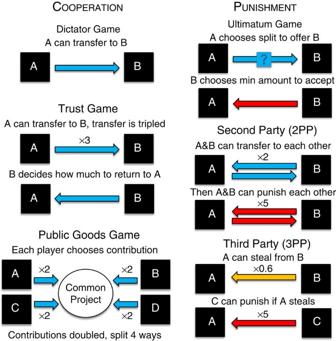Figure 1: The games used in our experiments. Economic games are commonly used to study cooperation (paying costs to benefit others) and punishment (paying costs to impose costs on others). Here we show the basic payoff structure of the cooperation and punishment games used in our experiments. Figure 1: The games used in our experiments. Economic games are commonly used to study cooperation (paying costs to benefit others) and punishment (paying costs to impose costs on others). Here we show the basic payoff structure of the cooperation and punishment games used in our experiments. Full size image We also include three decisions that involve norm-enforcing punishment: an Ultimatum Game (UG), a Prisoner’s Dilemma with second-party punishment (2PP) and a third-party punishment game (3PP) where the punisher is an impartial observer. In each of these decisions, players have the chance to pay a cost to impose a cost on someone behaving selfishly. See Fig. 1b for a description of each punishment game. Finally, we include a destructive (that is, negatively non-zero sum) competition decision: a two-player, sealed-bid All Pay Auction (AP) game. In the AP, each player chooses an amount to ‘invest’ in a competition over a prize. Any money spent is lost, but the player who spends more wins the monetary prize. If a cooperative phenotype exists, we would expect an individual’s play in the four cooperation decisions to be correlated. If the cooperative phenotype extends to norm enforcement and (non)-competitiveness, we would expect to see correlations between the cooperation games and the other measures. See Methods for experimental details. As a most straightforward analysis, we examine pairwise correlations between decisions in each game ( Fig. 2a ; Pearson’s correlation coefficient; all P -values are Bonferroni corrected to account for 28 simultaneous comparisons). We see that there are strong pairwise correlations among all of the cooperation decisions (PGG, DG, TG1, TG2; average magnitude=0.407, all P <0.0001). Similarly, there are significant, but less strong, pairwise correlations between norm-enforcing punishment decisions (2PP of defectors, 3PP of defectors, minimum acceptable offer (MAO) in the UG; average magnitude=0.231, all P <0.001). 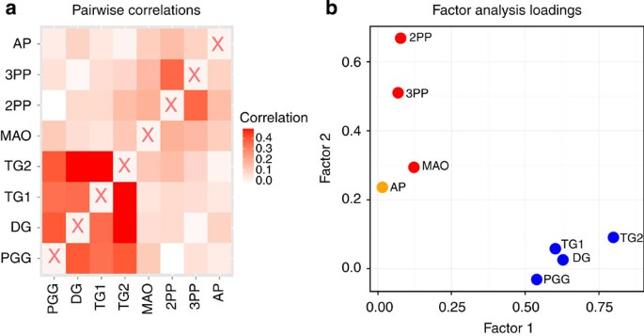Figure 2: A person’s play in one economic cooperation game is strongly related to play in other cooperation games, providing evidence for a cooperative phenotype. Furthermore, the cooperative phenotype does not extend to norm-enforcing punishment or to competition. (a) Pairwise correlation analyses using Pearson’s correlation coefficient show significant correlation patterns (after Bonferroni corrections) between decisions involving the choice to cooperate or defect (Dictator Game, Public Goods Game, Trust Game, both roles). There are also significant, but weaker, correlations between decisions to engage in norm-enforcing punishment (2PP, 3PP). However, there is little correlation between cooperation games and punishment games. Note that the correlation matrix is symmetric, such that entries above the diagonal are identical to the corresponding entries below the diagonal. (b) Factor analysis reveals a similar pattern—cooperation decisions load on one factor while norm-enforcing punishment decisions (2PP and 3PP) load on a second, orthogonal, factor. Similarly, competitiveness, as measured by the All Pay Auction, appears to be unrelated to cooperation and potentially weakly related to punishment. Data fromN=576 participants are analysed in both panels. Figure 2: A person’s play in one economic cooperation game is strongly related to play in other cooperation games, providing evidence for a cooperative phenotype. Furthermore, the cooperative phenotype does not extend to norm-enforcing punishment or to competition. ( a ) Pairwise correlation analyses using Pearson’s correlation coefficient show significant correlation patterns (after Bonferroni corrections) between decisions involving the choice to cooperate or defect (Dictator Game, Public Goods Game, Trust Game, both roles). There are also significant, but weaker, correlations between decisions to engage in norm-enforcing punishment (2PP, 3PP). However, there is little correlation between cooperation games and punishment games. Note that the correlation matrix is symmetric, such that entries above the diagonal are identical to the corresponding entries below the diagonal. ( b ) Factor analysis reveals a similar pattern—cooperation decisions load on one factor while norm-enforcing punishment decisions (2PP and 3PP) load on a second, orthogonal, factor. Similarly, competitiveness, as measured by the All Pay Auction, appears to be unrelated to cooperation and potentially weakly related to punishment. Data from N =576 participants are analysed in both panels. Full size image Conversely, we see no significant correlations (all P >0.2, most P >0.6) between norm-enforcement decisions and cooperation decisions, with the exception of a weak relationship between second-party punishment and positive reciprocity in the TG (2PP versus TG2; r= 0.15, P =0.033). This general lack of cross-correlation suggests that punishment and cooperation may be separate phenomena, rather than being driven by a common altruistic motivation. (The weak relationship between 2PP and TG2 hints at the possibility that positive and negative reciprocity may be related, but the lack of other correlations shows that punishment is not in general ‘altruistic’). We also see no significant correlations between any cooperation or punishment decisions and competitive behaviour in the auction (all P >0.50), except for a significant positive association between 2PP and AP ( r =0.15, P =0.027). See Supplementary Tables 1–3 and Supplementary Note 1 for additional correlation analyses. To examine the data in a more sophisticated way, we use factor analysis. Factor analysis is a statistical tool for reducing the dimensionality of a set of random variables (called features) by finding a simpler underling set of variables, called factors, that explain the correlation patterns found in the features (see Methods for a more detailed description). If there is a meaningful cooperative phenotype, we should find a single factor that explains the variance in the cooperation decisions of the PGG, DG, TG1 and TG2. If punishment or competition behaviours are related to the cooperative phenotype, we should see this factor also explain a portion of the variance in these behaviours. On the other hand, if behaviours in these different contexts are unrelated, we should either find that no underlying structure can simply summarize individual decisions, or that game behaviour is organized in a seemingly haphazard way. Performing factor analysis on our data reveals an underlying structure composed of two factors. These factors explain over 79% of the variance in the game decisions. As shown in Fig. 2b , we see that all cooperation behaviours (TG1, TG2, DG, PGG) load strongly on the first factor (all loadings>0.5), unlike the punishment games or the AP. Conversely, the norm-enforcing punishment decisions 2PP and 3PP load heavily (loadings>0.5) on the second, orthogonal factor, as does the UG-MAO and the AP decision, although somewhat more weakly (UG-MAO=0.29, AP=0.24). These analyses provide clear evidence in favour of a cooperative phenotype: Both the pairwise correlations and the factor analysis show that a thread of domain-general prosociality runs through our four cooperative game decisions. Note that we do not argue that these cooperation games are entirely driven by just that single motivation: for example, some games are influenced by expectations about others’ behaviour or preferences for reciprocity, equity and/or efficiency, while others are not. Our key result is that a substantial shared input to each of the cooperation decisions appears to be a domain-general trait of prosociality. Furthermore, neither punishment nor competitiveness appears to be related to cooperation in our data. This result suggests that the cooperative phenotype does not extend to these other social behaviours. This has important implications for our understanding of human psychology. Cooperation and punishment may not be two sides of the same coin, and being prosocial does not necessarily imply being averse to competition. Correlations between games and self-report measures Next we consider whether the cooperative phenotype we observe in these economic games extends to non-game measures. As a first step, we have our participants complete a survey of self-reported values and behaviours related to cooperation and punishment at the end of the experiment (see Methods and Supplementary Table 4 for details). 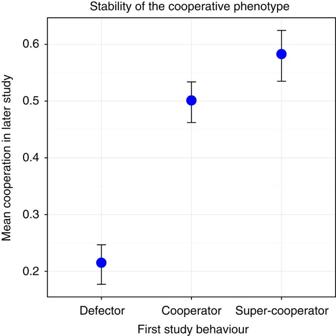Figure 4: The cooperative phenotype shows stability across time. AmongN=345 individuals who participated in multiple online studies, behaviour in the first study predicts behaviour in the last study (r=0.41; mean time between games=124 days). Here we visualize this correlation by showing the average cooperation in the last game based on play in the first game. We classify participants based on their play in the first game as defectors (who transfer nothing), cooperators (who transfer an intermediate amount) or super-cooperators (who makes the maximal transfer). Error bars indicate standard errors of the mean. We then ask how these cooperation and punishment self-report measures predict play in the cooperation and punishment games (linear regression with robust standard errors; P -values are Bonferonni corrected for four simultaneous comparisons). We find that play averaged over the four cooperation decisions is significantly positively correlated with responses averaged over the self-report cooperation measures ( P <0.001), but not the self-report punishment measures ( P =0.11; if anything, there is a negative but non-significant trend between game cooperation and punishment self-reports). Conversely, average play in the three norm-enforcing punishment decisions is significantly positively correlated with responses averaged over the self-report punishment measures ( P =0.008), and unrelated to the self-report cooperation measures ( P =0.68). These correlations are robust to extensive demographic controls (see Supplementary Table 5 ), and provide evidence that the cooperative phenotype extends beyond economic games. We also compare the relative strength of connection between games and self-report values versus self-report behaviours. To do so, we create separate subject-level averages for cooperation values, cooperation behaviours, punishment values and punishment behaviours, and repeat the two regressions above using these four separate independent variables (Bonferonni corrected for eight multiple comparisons). We see that it is cooperation values that are particularly correlated with cooperation game play rather than self-report cooperation behaviours, and that the relationship between punishment games and values/behaviour is weaker than that of the cooperation games (see Supplementary Table 6 ). Further evidence comes from examining pairwise correlations between game play and responses to each self-report question individually (including Bonferroni corrections for 70 multiple comparisons). Doing so finds that play averaged over the four cooperation games correlates significantly (Bonferroni-corrected Pearson’s correlation, P <0.05) positively with the values-related questions ‘I would support an increase in taxes if it were used to help the less well-off in society’ ( r =0.18), ‘People should be willing to help others who are less fortunate’ ( r =0.19), and ‘It is important to allow people you don’t know well to borrow items of some value such as dishes or tools’ ( r =0.16), and negatively with the reverse-coded values question ‘These days people need to look after themselves and not worry about others’ ( r =−0.21). The only significant correlation for play averaged over the three norm-enforcing punishment games was the self-reported frequency of ‘[Thinking] about how to get revenge on someone you had been angry at’ ( r =0.17). Correlations between cooperation games and actual helping Thus far we have provided evidence that play correlates across cooperation games, and that cooperation game play is correlated with moral values but not self-report behaviours. The lack of correlation we observe between cooperative game play and self-report cooperative behaviours may be driven by the inaccuracy of self-reporting on behaviours that are seen as socially desirable (for example, people may over-report being altruistic). Thus we conduct a second experiment to examine actual helping behaviour. We recruit another N =497 participants to play a PGG and a DG and take a brief demographic survey. After finishing the demographics survey, participants enter the ‘real-effort helping’ stage: they are told that the experiment is over, and are then given the option to help the experimenters by providing feedback on the instructions for a future experiment. It is repeatedly stressed that providing feedback is optional, and will not affect their earnings in this experiment or eligibility for future experiments. 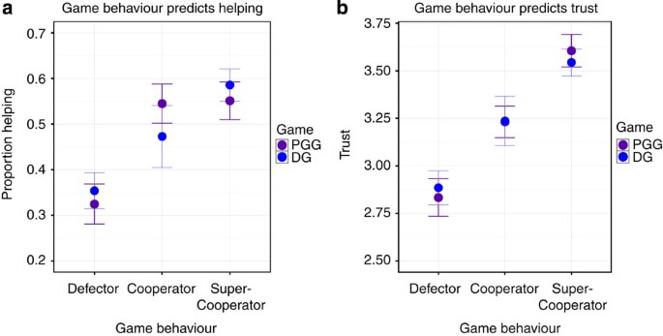Thus participants have the opportunity to engage in an actual helping task unrelated to the cooperation games, and that is not obviously part of an experiment. Figure 3: The cooperative phenotype extends to helping decisions involving real effort as well as generalized trust levels. (a) Cooperation in economic games predicts prosociality in a non-game helping task that is not obviously part of an experiment. Defectors (those who contribute 0 in the PGG/DG) are less likely to help than either cooperators (those who contribute more than 0 but less than the maximum) or super-cooperators (those who contribute the maximum amount). (b) Cooperators and super-cooperators also have higher generalized trust than defectors, as measured by a modified version of the trust question in the World Values Survey. Error bars indicate standard errors of the mean. Data fromN=497 participants analysed in both panels. Figure 3a shows a strong positive relationship between cooperation in the economic games and choosing to provide help (linear probability model with robust standard errors: PGG P <0.001, DG P =0.001, robust to demographic controls, see Supplementary Table 7 ; for visualization purposes only, we split participants into those who give nothing (‘defectors’), those who give the maximum amount (‘super-cooperators’) and those who give an intermediate amount (‘cooperators’)). These results provide evidence that the cooperative phenotype extends to actual helping behaviour beyond economic games. Figure 3: The cooperative phenotype extends to helping decisions involving real effort as well as generalized trust levels. ( a ) Cooperation in economic games predicts prosociality in a non-game helping task that is not obviously part of an experiment. Defectors (those who contribute 0 in the PGG/DG) are less likely to help than either cooperators (those who contribute more than 0 but less than the maximum) or super-cooperators (those who contribute the maximum amount). ( b ) Cooperators and super-cooperators also have higher generalized trust than defectors, as measured by a modified version of the trust question in the World Values Survey. Error bars indicate standard errors of the mean. Data from N =497 participants analysed in both panels. Full size image We also find that cooperation in the games predicts participants’ responses to an adapted version of a widely used question from the World Values Survey regarding generalized trust, in which we ask ‘How much do you agree with the statement: ‘Most people can be trusted.’?’ using a 5-point Likert Scale from ‘Completely disagree’ to ‘Completely agree’ ( Fig. 3b ; linear regression with robust standard errors: PGG P <0.001, DG P <0.001, robust to demographic controls, see Supplementary Table 8 ; note that on average defectors are below the mid-point on the scale, while cooperators and super-cooperators are above the mid-point). These results further demonstrate that economic games tap into a domain-general cooperative phenotype that extends beyond simple games. In addition, they are consistent with prior work relating trust and cooperative behavior [15] , [16] . Stability of game play over time We now turn from domain generality to stability over time: Does one’s cooperation behaviour today predict their cooperative behaviour in the future? Or is cooperation entirely dependent on context and situational effects? If the cooperative phenotype represents a general predisposition towards cooperation, then we would expect game play to be reasonably stable given the substantial degree of stability that has been shown for other personality traits (for example, the ‘Big Five’ [17] , [18] ). To test the stability of game play, we analyse the data from 15 cooperation studies run over a period of 2 years. Each study includes a cooperation game (Prisoner’s Dilemma, DG, TG or PGG) played online by participants from around the world, for stakes of between 40 cents and $1. As we are interested in both generalizability and stability across time, many of the games differ in their details (exact payoff structure, language of the instructions, and so on), but all decisions involve the option to increase the payoffs of others at a cost to oneself. See Methods for details. To assess stability, we analyse the behaviour of individuals who have participated in more than one experiment ( N =345). Specifically, we compare the play in the first and last decisions in the data set made by each of these individuals (mean time between first and last decisions=124 days). Cooperation in the first decision significantly predicts cooperation in the last decision ( Fig. 4 ; linear regression, coeff=0.389, P <0.001, Supplementary Table 9 col 1), and the correlation coefficient for cooperation games across time ( r =0.36) is similar to the average correlation across cooperation games played at the same time ( r =0.41). To help illustrate the strength of this relationship, we note that defectors (those who give nothing) in their first decision are over 60% likely to again give nothing in their last decision. Similarly, individuals who give the maximum amount in their first game (‘super-cooperators’) are over 40% likely to again be super-cooperators (and over 60% likely to cooperate at a non-zero level) in their last game. Furthermore, we see no evidence that the strength of the correlation between the first and last game declines as the time between the two games increases, indicating stability (interaction between first decision and months between decisions, P =0.473, Supplementary Table 9 col 2). Figure 4: The cooperative phenotype shows stability across time. Among N =345 individuals who participated in multiple online studies, behaviour in the first study predicts behaviour in the last study ( r =0.41; mean time between games=124 days). Here we visualize this correlation by showing the average cooperation in the last game based on play in the first game. We classify participants based on their play in the first game as defectors (who transfer nothing), cooperators (who transfer an intermediate amount) or super-cooperators (who makes the maximal transfer). Error bars indicate standard errors of the mean. Full size image Thus, the cooperative phenotype is not just domain general but also stable over time. In addition to demonstrating temporal stability, these results indicate that our cross-game correlation results reported above are not driven by consistency effects: even when measurements occur months apart, there is a high degree of correlation across games. Here we have presented a range of evidence in support of a ‘cooperative phenotype’: cooperation in anonymous, one-shot economic games reflects an inclination to help others that has a substantial degree of domain generality and temporal stability. The desire to pay costs to benefit others, so central to theories of the evolution and maintenance of cooperation, is psychologically relevant and can be studied using economic games. Furthermore, our data suggest that norm-enforcing punishment and competition may not be part of this behavioral profile: the cooperative phenotype appears to be particular to cooperation. Phenotypes are displayed characteristics, produced by the interaction of genes and environment. Though we have shown evidence of the existence (and boundaries) of the cooperative phenotype, our experiments do not illuminate whether cooperators are born or made (or something in between). Previous work has shown that cooperation varies substantially across cultures [19] , [20] , [21] , [22] , [23] , and is influenced by previous experience [24] , [25] , [26] , [27] , indicating an environmental contribution. On the other hand, a substantial heritable component of cooperative preferences has also been demonstrated [28] , [29] , as well as substantial prosocial behaviour and preferences among babies [30] , [31] and young children [32] , [33] . The ‘phenotypic assay’ for cooperation offered by economic games provides a powerful tool for future researchers to illuminate this issue, teasing apart the building blocks of the cooperative phenotype. Our finding that cooperation and punishment are not in general correlated has important implications for the study of human social behaviour. A wide range of evolutionary game theory models have explained the co-evolution of cooperation and punishment by assuming that these two traits are linked [34] , [35] , [36] , [37] . Our results suggest that these models should be revisited (for example, using models with expanded strategy sets where cooperation and punishment vary separately [38] , [39] , [40] , [41] , [42] , [43] ). The lack of correlation we find between cooperation and punishment is also consistent with previous work arguing that rejection of unfair offers in the UG (one particular form of punishment) is not prosocial by showing that UG rejections do not correlate with cooperation in various other games [44] . Our factor analysis suggests an even stronger conclusion: we find that UG rejection is in fact mostly distinct from both cooperation and norm-enforcing punishment. This finding highlights the psychological complexity involved in UG rejections, where the same behaviour can result from many motives (for example, fairness, spite or concern with relative standing) [45] , and cautions against using the UG as a general measure of prosocial preferences. Unlike the argument of ref. 44 , however, we do find some evidence of ‘strong reciprocity’ [46] , [47] in the positive correlation between the trustworthiness of Player 2 in the TG (positive reciprocity) and second-party punishment in the 2PP game (negative reciprocity). An important direction for future work examining the relationship between cooperation and punishment is to explore repeated games, rather than the one-shot games (without feedback) studied here. The dynamics of punishment can operate very differently in repeated games [48] , [49] , [50] , and thus different correlations with cooperation may be found in that context. Additionally, all of the studies presented here are correlational. The correlations we find between different cooperation games (and different punishment games) suggest that manipulations that alter play in one game should similarly affect play in other games. Recent work from our group provides evidence in support of this prediction: prior experience playing a series of short repeated Prisoner’s Dilemma games similarly decreases cooperation in a one-shot PGG, TG and DG, relative to prior experience with a series of long repeated Prisoner’s Dilemmas [27] . Future studies testing this prediction in additional domains will help to shed further light on the robustness of the cooperative phenotype. Our finding of strong within-individual correlations between play in our different cooperation games, as well as stability in cooperative play across time, is consistent with a previous study that found within-individual correlations in dyadic cooperation games played at different times by 108 Japanese participants [51] . We show that these correlations extend to the multi-player PGG, and a substantially larger sample of US residents. Another study, conversely, did not find significant within-subject correlations between play in a modified DG, PGG, UG and asynchronous Prisoner’s Dilemma (with the exception of play as the second mover in the Prisoner’s Dilemma, which correlated with all the other games) [52] ; this lack of significance may be due to lack of statistical power, however, as this study included only 61 participants. In more recent work, we have also demonstrated a correlation between play in a continuous Prisoner’s Dilemma and a DG [53] . Our stability results are consistent with previous work that showed that play in early rounds of a cooperation game was predictive of play later, demonstrating short-term temporal stability [54] . The correlation we demonstrate over the span of months shows that previous results were indeed driven by trait stability rather than by short-term consistency effects. Our results are also consistent with previous work showing stability in conditional cooperation preferences [55] ; we show a strikingly similar level of consistency in unconditional one-shot cooperation. The correlation we find between real effort cooperation and cooperation in economic games adds to a growing literature using cooperation games to predict pro-social behaviours in the field [56] , [57] , [58] . These findings also suggest that the lack of giving in a recent field version of the DG [59] was the result of some particular features of that scenario, rather than a general lack of external validity of economic games. More generally, examining the relationship between punishment in the lab and the field is an important direction for future work. Our results also offer powerful evidence for the value of small-stakes online experiments. Even though our games were conducted using the online platform Amazon Mechanical Turk [14] which necessarily involves less control than lab studies, and used smaller stakes (<$1) than is typical of most lab studies [60] , we still find both generality and stability. Future work should test the extent to which our findings using this online subject pool generalize to more traditional laboratory pools, as well as cross-cultural experiments. Cooperation is central to the success of human societies, and therefore understanding how to promote cooperation is a central challenge for humankind. Our demonstration of the domain generality of play in economic games suggests that these games are indeed useful tools for exploring cooperation, and provides support for the central assumption underlying most theoretical work on the evolution of cooperation. General experimental design All of our experiments are conducted via the internet. Specifically, participants living in the United States are recruited using the online labour market Amazon Mechanical Turk (AMT), and redirected to an external website where our experiment is implemented. AMT is an online labour market where employers contract with workers to complete short tasks for relatively small amounts of money. Workers are paid a fixed baseline wage (show-up fee for experiments) plus an additional variable bonus (which can be conditioned on their performance). All participants provide informed consent, and this work has been approved by the Harvard University Committee on the Use of Human Subjects. AMT and other online platforms are extremely powerful tools for conducting experiments, allowing researchers to easily and cheaply recruit a large number of participants who are substantially more diverse than typical college undergraduates. Nonetheless, there are potential issues in online experiments that either do not exist in the physical laboratory, or are more or less extreme (see ref. 14 for a detailed discussion). Most notably, experimenters have substantially less control in online experiments, as participants cannot be directly monitored the way they are in the traditional lab. Thus, multiple people might be working together as a single participant, or one person might log on as multiple participants simultaneously (although AMT goes to great lengths to prevent multiple accounts, and, based on IP address monitoring, it happens only rarely). One might also be concerned about the representativeness of participants recruited through AMT, although they are substantially more demographically diverse than participants in the typical college undergraduate samples. To address these potential concerns, numerous recent studies have explored the validity of data gathered using AMT (for an overview, see ref. 61 ). Most relevant here are two direct replications using economic games, demonstrating quantitative agreement between behaviour in the physical lab and on AMT with approximately 10-fold lower stakes in a repeated PGG [62] and a one-shot Prisoner’s Dilemma [14] . It has also been shown that play in one-shot PGGs, TGs, DGs and UGs on MTurk using $1 stakes is in accordance with behaviour in the traditional laboratory [60] . The present paper adds further evidence of the reliability of AMT data, by showing internal validity (via correlations between similar games in Experiment 1), external validity (via correlations between games and related moral values in Experiment 1, as well as actual helping behaviour in Experiment 2), and stability. Experiment 1: Correlations between games and self-report measures We recruit 576 individuals to participate in Experiment 1. Participants earn 50 cents for accepting our online survey. They then make decisions in a number of economic games (as described below in more detail). After completing the study, one role in one of these games is chosen at random, participants are matched accordingly and then paid based on their earnings in that game (up to $2, depending on which game is picked and what the players’ decisions are). This payment method prevents ‘portfolio building’ and encourages participants to play each game as if it were the only decision that would count in the experiment. Participants are informed of this payment scheme and no deception is used. The entire experiment takes between 10 and 17 min. Each game has the following form: first, individuals read the rules of the game; next they answer a comprehension question about the rules; and finally they enter their decisions for each potential player role. We find that the average participant answers 93% of comprehension questions correctly, and our analyses exclude the 7% of decisions in which comprehension was failed. We also note that 72% of individuals answer every single comprehension question correctly. After playing the games, participants answer questions about how often they engage in certain behaviours, questions about their social values and finally a demographics questionnaire. We use a number of economic games in our experiment. Each of the games is played for points, which are converted to dollars at the rate of 1.5 cents per point. We include three games that involve paying a cost to give a benefit to one or more others (that is, fit the definition of ‘one-shot cooperation’): In the PGG, 4 participants start with 100 points each and choose to contribute any amount (0 to 100 points) to a common project. Anything contributed to the common project is doubled and split among the group. In the TG, 2 players each start with 50 points. Player 1 (TG1, or the Trustor) chooses whether to transfer their 50 points to player 2 (TG2, the Trustee). If TG1 chooses to transfer, the points are tripled and given to TG2. TG2 can then choose to transfer back any fraction of this amount to TG1 (0 to 150 points). In the DG, one participant (the Dictator) starts with 100 points and unilaterally chooses how much (0 to 50 points) to give to a passive recipient. In each of these games, a higher choice entails the decider incurring a larger cost while one or more others receive a larger benefit (although note that, in the case of TG1, a higher choice may result in higher earnings depending on the choice of TG2). We also include three games that involve paying a cost to impose a cost on another (that is, punishment): In the UG, one player (the Proposer) is given a 100-point endowment to split with the second player (the Responder). The Proposer makes a single take-it-or-leave-it offer to the responder of X points (0 to 50). If the Responder accepts the offer, they receive X points and the Proposer receives 100− X points. If the Responder rejects the offer, both individuals receive 0 points. Rather than responding to a specific offer, responders indicate their minimal acceptable offer (MAO), such than an offer below the MAO will be rejected. In the Second Party Punishment (2PP) game, two individuals play a Prisoner’s Dilemma game: they each begin with 100 points, and then choose whether to give up 30 points to give 60 points to the other (C), or not (D). After making their C/D decision, they advance to a second stage, in which they can pay up to 14 points to reduce the other player’s payoff (each cent spent reduces the other’s payoff by 5). Punishment decisions are made using the strategy method: rather than being informed of the other player’s choice, participants indicate (i) the amount to punish if the other cooperated, and (ii) the amount to punish if the other defected. We take punishment of defection as our measure of norm-enforcing 2PP. In the Third-Party Punishment (TPP) game, two players are each endowed with 100 points. Player A can then choose whether to ‘take’ from Player B. If A takes, then Player B loses 50 points while A gains 30 points (thus theft is inefficient, and it is socially optimal to not steal; this part of the game is analogous to a unilateral Prisoner’s Dilemma). A third player, Player C, then receives 20 points and chooses how many to pay to reduce Player A’s payoff if Player A chooses ‘take’, with each point spent reducing Player A’s payoff by 5 points. We take points spent by Player C as our measure of 3PP. We note that the 2PP and 3PP game formulations used here are somewhat non-standard: 2PP uses a two-player Prisoner’s Dilemma followed by punishment, rather than the more typical four-player PGG with punishment [63] , [64] , and 3PP uses a taking frame as in ref. 65 , rather than the more traditional giving frame [66] , [67] . Nonetheless, both games capture the phenomenon of norm-enforcing punishment, and successfully elicit substantial variance in levels of such punishment (as shown below in Supplementary Fig. 1 ). Therefore the lack of correlation observed between cooperation and punishment is not due to an overall lack of punishment behaviour. Finally, we include an economic game designed to measure competitiveness: the All-Pay Auction (AP). In the AP, two individuals are given an endowment of 100 points. They choose how much to spend to compete to win a 100-point prize. The individual who invests more receives the 100 points (if both players invest equally, one is chosen at random to receive 100 points). However, any money spent by either player is lost. The games are presented in random order and each participant makes a decision for each possible player role in each game using the strategy method. The distribution of play in each decision of each game is shown in Supplementary Fig. 1 , and the instructions for each game are given in the Supplementary Methods . Following the games, subjects complete 35 self-report questions regarding cooperation and punishment outside of the laboratory. Some of these questions are about endorsement of social values related to either cooperation or punishment, and others are about engaging in either cooperation or punishment behaviours. Some of these questions are slightly modified versions of questions used in the cross-cultural literature, collected from the World Values Survey and the General Social Survey; others are generated specifically for this study. Supplementary Table 4 gives a list of all of the self-report questions collected. Game factor analysis In addition to the pairwise correlation analysis of Fig. 2a , we use a more structural approach to look for relationships between play in the different games of Experiment 1. To do so, we apply factor analysis (FA). We sketch the basic technique of FA here, and refer the reader interested in more technical coverage to other work [68] . The structural model underlying factor analysis makes the following assumptions: we assume that we have an n -dimensional linear space of features (labeled x 1 , …, x n ). Here, the features are behaviours in each of our economic games. We assume that the feature space is actually ‘too large’—that is, features are actually linear combinations of attributes from a smaller-dimensional factor space (labeled f 1 , f 2 , .., f k ). So an individual with factor vector f will have a level of feature x i given by x i = a i * f , where a i is some constant vector of weights. In our example, a potential set of factors is given by an individual-specific propensity to cooperate and propensity to punish, which are then expressed in the economic games. We observe features (with normally distributed measurement error) for n individuals, but not underlying factors. The statistical problem that FA solves is to use the observed features to figure out both the dimension of the underlying factor space and the inverse mapping between observed values of features for each individual and actual underlying factor values for each individual. Based on our correlational results that demonstrate two main clusters of inter-game correlations (cooperation games and punishment games), we hypothesize a two-dimensional factor space. Indeed, performing FA shows that two factors explain >79% of the variance in features, and that none of the remaining six factors explains a substantial amount of variance (the next most informative factor explains only 7.5% of the variance). We therefore use two factors and apply varimax rotation to recover interpretable loadings for the factors (results shown in Fig. 2b ). Experiment 2: Real-effort helping In Experiment 2, we recruit N =497 individuals to perform the following three-stage experiment. The first stage of the experiment is a one-shot PGG played in groups of four. Participants are endowed with 40 cents and asked how much they wish to keep for themselves versus contribute to a group pot. Every cent that is contributed to the group pot is doubled and split evenly among the four group members. To assess their understanding of the payoff structure, participants are asked two comprehension questions about the rules of the PGG. To avoid contamination between stages, participants are not informed about the outcome of Stage 1 until receiving their payment after the conclusion of the study. The second stage is a DG. Participants are endowed with another 40 cents and choose how much to give to another person (not a member of the participant’s PGG group). Participants then complete a brief demographic survey, including a question regarding generalized trust, in which participants are asked ‘How much do you agree with the statement: ‘Most people can be trusted.’?’ using a 5-point Likert Scale from ‘Completely disagree’ to ‘Completely agree’. After finishing the demographics survey, participants enter the third stage. They are not informed that this stage is part of the experiment. Instead, they are informed that the study is over, but that the experimenters are in the process of setting up additional studies for other participants and are unsure about whether the instructions for these studies are clear. Participants are then asked if they would like to aid the experimenters by proofreading several paragraphs of instructions (without compensation). It is repeatedly stressed that this proofreading is optional, and that their choice will not affect their earnings in this experiment or eligibility for future experiments. Participants who choose to help the experimenters are then shown a set of instructions and asked from comments. The exact wording of this third stage is shown in the Supplementary Methods . We use willingness to accept the proofreading task as our measure of real-effort helping. Experiment 3: Stability of game play over time To assess the stability of game play, we aggregate 15 cooperation game studies that our lab conducted on AMT between early 2011 and summer 2013, and examine the play of individuals who participated in more than one experiment. Eleven of these studies are previously unpublished; four have been published [14] , [24] , [69] , [70] and are re-analysed here. Each of these 15 studies includes a cooperation game (Prisoner’s Dilemma, DG, TG or PGG) played by participants for stakes of between 40 cents and $1. We do not include any games to which a secondary manipulation (for example, priming, time pressure, addition of punishment, and so on) is applied. Instead, we pool baseline experiments with control conditions from studies that do include such manipulations (although some of the games do include minor changes in the framing, for example, a PGG framed as extraction from a common resource instead of adding to a common project). Across the 15 studies, we find 345 individuals who participated more than once (from a total potential set of 3,415 individuals who participated in these 15 studies). Unique individuals are identified by their AMT WorkerID, which Amazon goes to lengths to ensure represents a single individual (among other things, each WorkerID must be linked to a unique bank account). To look for stability of behaviour across time we normalize all cooperation decisions such that the maximum possible transfer has value 1. We then ask how each individual’s decision in the first of their games in the data set predicts their play in the last of their games. How to cite this article: Peysakhovich, A. et al . Humans display a ‘cooperative phenotype’ that is domain general and temporally stable. Nat. Commun. 5:4939 doi: 10.1038/ncomms5939 (2014).